NEDD4 controls intestinal stem cell homeostasis by regulating the Hippo signalling pathway The Hippo pathway plays crucial roles in regulating organ size and stem cell homeostasis. Although the signalling cascade of the core Hippo kinases is relatively well understood, little is known about the mechanisms that modulate the activity of the Hippo pathway. Here, we report identification of NEDD4, a HECT-type E3 ubiquitin ligase, as a regulatory component of the Hippo pathway. We demonstrate that NEDD4 ubiquitylates and destabilizes WW45 and LATS kinase, both of which are required for active Hippo signalling. Interestingly, MST1 protects WW45, but not LATS2, against NEDD4. We also provide evidence indicating that NEDD4 inactivation at high cell density is a prerequisite for the elevated Hippo activity linked to contact inhibition. Moreover, NEDD4 promotes intestinal stem cell renewal in Drosophila by suppressing Hippo signalling. Collectively, we present a regulatory mechanism by which NEDD4 controls the Hippo pathway leading to coordinated cell proliferation and apoptosis. Determination and maintenance of the proper organ size are of paramount importance in all living organisms. The Hippo pathway represents one of the crucial mechanisms in control of organ size via modulating cell proliferation and apoptosis. Most of the Hippo signalling components were initially identified from genetic studies in Drosophila melanogaster [1] , [2] , [3] . Specifically, WW domain containing scaffold protein Salvador (Sav), Ste-20 family kinase Hippo (Hpo), NDR kinase Warts (Wts) and transcription co-activator Yorkie (Yki) are core components of the Hippo pathway in Drosophila [4] , [5] , [6] . Sav forms a complex with Hpo and Wts through its C-terminal Sav-Rassf-Hpo (SARAH) domain and WW domains, respectively, and the trimeric interaction facilitates phosphorylation and activation of Wts by Hpo [6] , [7] . Activated Wts phosphorylates Yki and phosphorylated Yki is subsequently sequestered in the cytoplasm through interaction with the 14-3-3 protein. Inactivation of Yki leads to decreased expression of the cell cycle regulator Cyclin E and the Drosophila inhibitor of apoptosis protein DIAP1 (refs 8 , 9 ). The Hippo signalling cascade and core components are highly conserved from Drosophila to mammals (Sav for WW45 or SAV1, Hpo for MST1/2, Wts for LATS1/2, and Yki for YAP and TAZ in mammals, respectively), and mammalian homologues are able to rescue the overgrowth phenotype of Drosophila mutants [6] , [10] , [11] . It has recently been reported that the mammalian Hippo pathway regulates cell-to-cell contact inhibition as well as organ size [12] , [13] , [14] , [15] . Thus, dysregulation of the mammalian Hippo pathway is linked to tumorigenesis. Core Hippo components, MST1/2 , LATS1/2 and WW45 , are either hypermethylated or mutated in various tumours and cancer cells [1] , [16] , [17] . YAP is elevated in some human cancers, including breast, liver and colorectal cancer, and this overexpression leads to inhibition of apoptosis and enhancement of the epithelial–mesenchymal transition as well as anchorage-independent growth [18] , [19] , [20] . Several lines of evidence also indicate that the Hippo signalling modulates homeostatic self-renewal and regeneration of intestinal stem cells (ISCs) [21] , [22] . Although the signalling cascade of the core kinase pathway is relatively well understood, much less is known about the regulatory mechanisms that fine-tune the Hippo pathway. Given that Sav proteins become stable in Drosophila when the 26S proteasome is inhibited and Wts protein levels are post-transcriptionally regulated [7] , [23] , it is plausible that the ubiquitin-proteasome system plays a role in regulating the Hippo pathway. Ubiquitin-activating (E1), conjugating (E2) and ligating (E3) enzymes work in concert to accomplish protein ubiquitylation. Among these, members of the E3 ubiquitin (Ub) ligase family confer substrate specificity by binding substrate proteins [24] . NEDD4 (neural precursor cell expressed, developmentally down-regulated protein 4; also known as NEDD4-1) is an E3 Ub-ligase composed of a N-terminal C2 domain, four WW domains that bind to PY motifs (L/PPXY) and a C-terminal HECT (Homologous to E6-AP carboxyl terminus) domain [25] . The C2 domain is crucial for Ca 2+ -dependent plasma membrane localization of NEDD4 (refs 26 , 27 ). NEDD4 is known to positively regulate cell proliferation and growth. This is supported by the observation that the NEDD4 knockout (KO) mouse shows apparent growth retardation compared with wild-type littermates and that NEDD4 KO mouse embryonic fibroblast cells grow slowly. Such phenotypic outcomes originate from the NEDD4-mediated positive regulation of IGF-1 and insulin signalling [28] . It has recently been reported that NEDD4 family member proteins, including ITCH [29] , [30] and NEDD4 (ref. 31 ), negatively regulate LATS1, suggesting that NEDD4 plays a role in Hippo signalling. In the present study, we report the role of NEDD4 as a key regulator of the Hippo signalling pathway. NEDD4 negatively regulates the stability of WW45 and LATS kinase, which leads to alterations in cell proliferation and ISC homeostasis. NEDD4 directly interacts with WW45 To understand how the Hippo signalling pathway is controlled, we set out to identify a specific regulator using affinity purification combined with mass spectrometry. WW45 was chosen as the bait since WW45 is the sole adaptor protein that makes a core complex with MST1/2 and LATS1/2. We thus expressed FLAG-WW45 in HEK293T cells and performed affinity purification. Subsequent liquid chromatography-mass spectrometry analysis revealed several WW45-interacting proteins. Specifically, our mass spectrometry data showed that WW45-immunoprecipitates contained MST1 and LATS2, both of which are known to interact with WW45, as well as a novel interacting protein, NEDD4 E3 Ub-ligase ( Fig. 1a ). We confirmed the in vivo interaction between WW45 and NEDD4 using both transiently expressed and endogenous proteins in HEK293T cells ( Supplementary Fig. 1a and Fig. 1b ). We performed an in vitro pulldown assay using GST-WW45 purified from Escherichia coli and immunopurified FLAG-NEDD4 proteins. NEDD4 was readily detected in the fractions eluted from the GST-WW45 affinity column but not in eluates from the glutathione S -transferase (GST) column, indicating that the interaction between these proteins was direct ( Fig. 1c ). Next, we constructed N- and C-terminal-truncated WW45 mutants (199C N198, and N321) to map the binding region for NEDD4. Whereas WW45 interacts with its binding partners mostly through either the WW domains or the SARAH domain [6] , it bound to NEDD4 via its N-terminal region ( Fig. 1d ). We also constructed several NEDD4 deletion mutants and found that the very N-terminus (amino acids 1-100) was crucial for binding to WW45 ( Fig. 1e and Supplementary Fig. 1b ). Taken together, NEDD4 is a newly identified WW45-interacting protein and they interact with each other directly through their N-terminal regions. 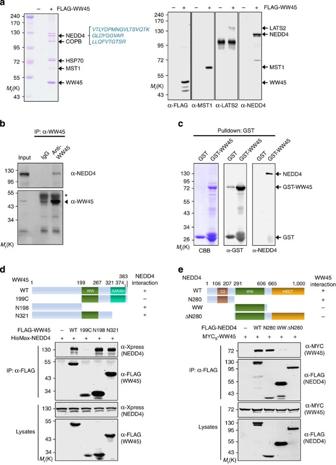Figure 1: NEDD4 is a new WW45-interacting protein. (a) WW45-interacting proteins were identified. Either mock- or FLAG-WW45-transfected HEK293T cells were immunoprecipitated with anti-FLAG M2 resin. Cells were pre-treated with 20 μM MG132 for 4 h. Immunoprecipitates were separated by SDS–polyacrylamide gel electrophoresis and subjected to coomassie blue staining or immunoblotting with indicated antibodies. Peptide sequences of NEDD4 detected from the analysis of mass spectrometry are shown. (b) WW45 and NEDD4 are endogenously associated with each other. Immunoprecipitation (IP) with IgG or anti-WW45 antibody was performed with HEK293T lysates treated with 20 μM MG132 for 4 h and analysed by immunoblotting with indicated antibodies. Asterisk and arrowhead designate IgG and immunoprecipitated WW45, respectively. (c) NEDD4 directly interacts with WW45in vitro. Purified FLAG-NEDD4 and either GST or GST-WW45 were incubated with glutathione sepharose for 1 h. Precipitates were analysed by immunoblotting. (d) The N-terminus of WW45 is important for interaction with NEDD4. HisMax-NEDD4 was co-transfected with various FLAG-WW45 deletion mutants (WT, wild-type; 199C, N-terminal deletion; N198 and N321, C-terminal deletion, amino acids (a.a.) 1–198 and a.a. 1–321 region, respectively) in HEK293T cells. At 24 h post transfection, cells were treated with 20 μM MG132 for 4 h. Cell lysates were immunoprecipitated with anti-FLAG M2 resin and immunoblotted with indicated antibodies. (e) N-terminus of NEDD4 is required for association with WW45. MYC9-WW45 was co-transfected with various FLAG-NEDD4 constructs (WT, wild-type; N280, a.a. 1–280; WW, a.a. 281–620; ΔN280, a.a. 281–1000) in HEK293T cells. At 24 h post transfection, cells were treated with 20 μM MG132 for 4 h. Cell lysates were immunoprecipitated with anti-FLAG M2 resin and immunoblotted with indicated antibodies. Figure 1: NEDD4 is a new WW45-interacting protein. ( a ) WW45-interacting proteins were identified. Either mock- or FLAG-WW45-transfected HEK293T cells were immunoprecipitated with anti-FLAG M2 resin. Cells were pre-treated with 20 μM MG132 for 4 h. Immunoprecipitates were separated by SDS–polyacrylamide gel electrophoresis and subjected to coomassie blue staining or immunoblotting with indicated antibodies. Peptide sequences of NEDD4 detected from the analysis of mass spectrometry are shown. ( b ) WW45 and NEDD4 are endogenously associated with each other. Immunoprecipitation (IP) with IgG or anti-WW45 antibody was performed with HEK293T lysates treated with 20 μM MG132 for 4 h and analysed by immunoblotting with indicated antibodies. Asterisk and arrowhead designate IgG and immunoprecipitated WW45, respectively. ( c ) NEDD4 directly interacts with WW45 in vitro . Purified FLAG-NEDD4 and either GST or GST-WW45 were incubated with glutathione sepharose for 1 h. Precipitates were analysed by immunoblotting. ( d ) The N-terminus of WW45 is important for interaction with NEDD4. HisMax-NEDD4 was co-transfected with various FLAG-WW45 deletion mutants (WT, wild-type; 199C, N-terminal deletion; N198 and N321, C-terminal deletion, amino acids (a.a.) 1–198 and a.a. 1–321 region, respectively) in HEK293T cells. At 24 h post transfection, cells were treated with 20 μM MG132 for 4 h. Cell lysates were immunoprecipitated with anti-FLAG M2 resin and immunoblotted with indicated antibodies. ( e ) N-terminus of NEDD4 is required for association with WW45. MYC 9 -WW45 was co-transfected with various FLAG-NEDD4 constructs (WT, wild-type; N280, a.a. 1–280; WW, a.a. 281–620; ΔN280, a.a. 281–1000) in HEK293T cells. At 24 h post transfection, cells were treated with 20 μM MG132 for 4 h. Cell lysates were immunoprecipitated with anti-FLAG M2 resin and immunoblotted with indicated antibodies. Full size image NEDD4 ubiquitylates and destabilizes WW45 To determine the functional significance of the NEDD4–WW45 interaction, we tested whether NEDD4 affects the cellular level of WW45. We found that WW45 levels varied inversely with the levels of co-transfected NEDD4 ( Fig. 2a ). Moreover, NEDD4-mediated destabilization of WW45 was blocked by the proteasome inhibitor MG132. Co-expression of NEDD4 C967S , which lacks ubiquitin ligase activity owing to the replacement of Cys 967 with Ser [32] , and N-terminal deletion mutant NEDD4 ΔN280 did not affect WW45 levels, indicating that both the substrate-binding and E3 catalytic activity of NEDD4 were required for WW45 destabilization ( Fig. 2b ). Furthermore, ectopic expression of NEDD4 led to downregulation of endogenous WW45 ( Supplementary Fig. 2a ), which was also confirmed by a cycloheximide (CHX) chase assay ( Supplementary Fig. 2b ). To investigate whether endogenous NEDD4 contributes to the regulation of WW45, we depleted endogenous NEDD4 in HEK293T cells using RNA interference (RNAi). All three short interfering RNAs (siRNAs) against NEDD4 (si NEDD4 #1, si NEDD4 #2 and si NEDD4 #3) reduced NEDD4 levels and increased WW45 levels accordingly ( Fig. 2c ). This is also confirmed by the CHX chase assay with siRNAs that the halflife of WW45 was not declined in the presence of si NEDD4 , but not either si Scr or si ITCH as a control ( Supplementary Fig. 2c ). Next, we investigated whether NEDD4 mediates the proteasomal degradation of WW45 by its ubiquitylation. GST-WW45 purified from E. coli was ubiquitylated in vitro upon incubation with bacteria-expressed His-NEDD4 ( Fig. 2d ). To examine whether NEDD4 promotes ubiquitylation of WW45 in vivo , MYC 9 -WW45 was co-expressed in HEK293T cells with FLAG-NEDD4 vectors (NEDD4 WT , NEDD4 C967S or NEDD4 ΔN280 ). WW45 was extensively ubiquitylated by NEDD4 WT , but barely ubiquitylated in the presence of either NEDD4 C967S or NEDD4 ΔN280 ( Fig. 2e ). Endogenous WW45 ubiquitylation by NEDD4 was also validated with si NEDD4 ( Supplementary Fig. 2d ). Despite the major effect of NEDD4 on the ubiquitylation status of WW45, total cellular ubiquitin conjugates were not affected by the overexpression or knockdown (KD) of NEDD4. Taken together, these results demonstrate that NEDD4 directly binds to and ubiquitylates WW45, resulting in its proteasomal degradation. 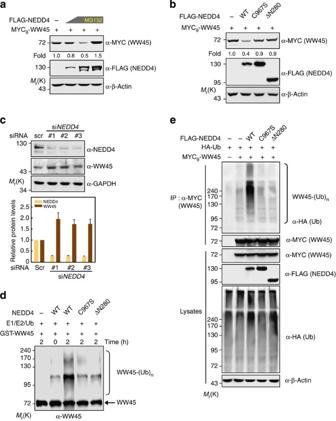Figure 2: NEDD4 negatively regulates WW45 stability as the specific E3 ubiquitin ligase. (a) NEDD4 decreases WW45 protein levels in a dose-dependent manner. HEK293T cells were transfected with MYC9-WW45 (0.5 μg) and FLAG-NEDD4 (0, 0.5, 2 μg), and treated with 20 μM MG132 for additional 4 h at 24 h post transfection as indicated. WW45 protein levels were quantitated by ImageJ and normalized to β-actin protein levels. (b) Both E3 Ub-ligase activity and direct interaction of NEDD4 are necessary for the regulation of WW45 protein levels. Only NEDD4WTis able to destabilize WW45. Neither NEDD4C967Snor NEDD4ΔN280mutant affects WW45 stability. MYC9-WW45 was co-transfected with FLAG-NEDD4 WT, -C967S or -ΔN280 mutant into HEK293T cells. WW45 protein levels were quantitated by ImageJ and normalized to β-actin protein levels. (c) NEDD4 knockdown stabilizes WW45. HEK293T cells were transfected with Scrambled (scr) or NEDD4-specific siRNAs. NEDD4 and WW45 protein levels were quantitated by ImageJ and normalized to glyceraldehyde 3-phosphate dehydrogenase (GAPDH) protein levels. Data represent mean±s.e.m. of four independent experiments. (d) NEDD4 ubiquitylates WW45in vitro. Purified GST-WW45 proteins were ubiquitylated in the presence of purified His-NEDD4in vitro. See Methods for further details. Afterin vitroubiquitylation reaction, samples were analysed by immunoblotting with anti-WW45 antibody. (e) NEDD4 ubiquitylates WW45in vivo. MYC9-WW45, HA-Ubiquitin and FLAG-NEDD4 were co-transfected into HEK293T cells as indicated and treated with MG132 (20 μM) for 4 h before harvest. Cell lysates were immunoprecipitated with anti-MYC (9E10) resin and analysed by immunoblotting with indicated antibodies. Figure 2: NEDD4 negatively regulates WW45 stability as the specific E3 ubiquitin ligase. ( a ) NEDD4 decreases WW45 protein levels in a dose-dependent manner. HEK293T cells were transfected with MYC 9 -WW45 (0.5 μg) and FLAG-NEDD4 (0, 0.5, 2 μg), and treated with 20 μM MG132 for additional 4 h at 24 h post transfection as indicated. WW45 protein levels were quantitated by ImageJ and normalized to β-actin protein levels. ( b ) Both E3 Ub-ligase activity and direct interaction of NEDD4 are necessary for the regulation of WW45 protein levels. Only NEDD4 WT is able to destabilize WW45. Neither NEDD4 C967S nor NEDD4 ΔN280 mutant affects WW45 stability. MYC 9 -WW45 was co-transfected with FLAG-NEDD4 WT, -C967S or -ΔN280 mutant into HEK293T cells. WW45 protein levels were quantitated by ImageJ and normalized to β-actin protein levels. ( c ) NEDD4 knockdown stabilizes WW45. HEK293T cells were transfected with Scrambled (scr) or NEDD4-specific siRNAs. NEDD4 and WW45 protein levels were quantitated by ImageJ and normalized to glyceraldehyde 3-phosphate dehydrogenase (GAPDH) protein levels. Data represent mean±s.e.m. of four independent experiments. ( d ) NEDD4 ubiquitylates WW45 in vitro . Purified GST-WW45 proteins were ubiquitylated in the presence of purified His-NEDD4 in vitro . See Methods for further details. After in vitro ubiquitylation reaction, samples were analysed by immunoblotting with anti-WW45 antibody. ( e ) NEDD4 ubiquitylates WW45 in vivo . MYC 9 -WW45, HA-Ubiquitin and FLAG-NEDD4 were co-transfected into HEK293T cells as indicated and treated with MG132 (20 μM) for 4 h before harvest. Cell lysates were immunoprecipitated with anti-MYC (9E10) resin and analysed by immunoblotting with indicated antibodies. Full size image NEDD4 associates with and destabilizes LATS kinase Because WW45 is a key component of the Hippo pathway and thereby regulates apoptotic processes, we investigated whether NEDD4 is able to control apoptosis through WW45. When NEDD4 was depleted by si NEDD4 in HEK293T cells, apoptosis was induced and further augmented by the treatment of an apoptosis-inducing drug, staurosporine (STS; Fig. 3a ). However, simultaneous KD of both NEDD4 and WW45 reversed STS-induced cell death albeit partially compared with what was seen with NEDD4 KD alone (the efficacy of sh WW45 is shown in Supplementary Fig. 3a ). It was also validated by the amount of cleaved poly [ADP-ribose] polymerase (PARP) and fluorescence-activated cell sorting analysis ( Fig. 3b and Supplementary Fig. 3b,c ). These results possibly suggested that NEDD4 might act on additional targets besides WW45 protein. Intriguingly, we noticed that NEDD4 depletion stabilized not only WW45 but also LATS2 ( Fig. 3b ). This is in agreement with the observation that protein levels for both LATS2 and WW45 were enhanced by the treatment of MG132 ( Fig. 3c and Supplementary Fig. 3d ). Thus, it is plausible that NEDD4 may also regulate LATS2 as its specific E3 Ub-ligase. Co-immunoprecipitation assays showed that NEDD4 bound to LATS2 mostly through amino acids 281–660 region that encompass the WW domains ( Fig. 3d and Supplementary Fig. 3e ). Furthermore, LATS2 protein levels were decreased by NEDD4 WT in a dose-dependent manner and recovered by MG132 treatment, whereas unaffected by the NEDD4 C967S mutant ( Fig. 3e and Supplementary Fig. 3f ). CHX chase assay also validated that LATS2 stability was rapidly decreased in the presence of NEDD4 ( Supplementary Fig. 3g ). In contrast to WW45, both NEDD4 WT and NEDD4 ΔN280 mutant were able to destabilize LATS2 ( Fig. 3 f ) as NEDD4 ΔN280 can bind to LATS2 but not to WW45. Moreover, LATS2 was polyubiquitylated in vitro ( Supplementary Fig. 3h ) and in vivo ( Fig. 3g ) by NEDD4 WT but not by NEDD4 C967S mutant. We also showed that NEDD4 was able to destabilize LATS1, another mammalian homologue of Drosophila Warts ( Supplementary Fig. 3i ). Taken together, these data indicate that NEDD4 negatively regulates LATS1 and LATS2 as well as WW45. 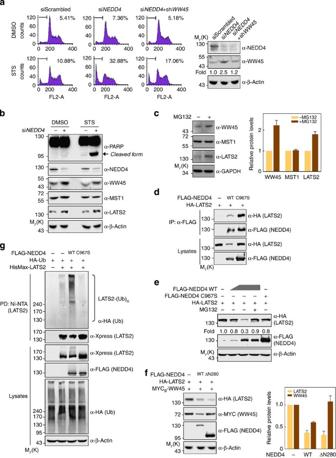Figure 3: LATS kinase is another substrate of NEDD4. (a) NEDD4 knockdown enhances staurosporine (STS)-induced apoptosis. HEK293T cells were transfected with NEDD4 siRNA alone or in conjunction with WW45 short hairpin RNA as indicated. At 48 h post transfection, cells were treated with 0.5 μM STS for 12 h before harvest. Cells were then collected for the FACS analysis to determine sub-G1 content or subjected to immunoblotting. WW45 protein levels were quantitated by ImageJ and normalized to β-actin protein levels (n=3). (b) WW45 and LATS2 are stabilized when NEDD4 expression is suppressed. Either scrambled siRNA or siNEDD4-transfected HEK293T cells were treated with STS (0.5 μM) for 12 h before harvest. Lysates were then analysed by immunoblotting with indicated antibodies. (c) WW45 and LATS2, but not MST1, are stabilized by MG132. HEK293T cells were treated with 20 μM MG132 for 4 h as indicated. WW45, MST1 and LATS2 protein levels were quantitated by ImageJ, normalized to β-actin levels and the relative protein levels are shown (n=4). (d) NEDD4 interacts with LATS2in vivo. HA-LATS2 was transfected with either FLAG-NEDD4 WT or C967S in HEK293T cells as indicated. Cell lysates were immunoprecipitated with anti-FLAG M2 resin and analysed by immunoblotting with indicated antibodies. (e) NEDD4 decreases LATS2 protein levels in a dose-dependent manner. HA-LATS2 was co-transfected with either FLAG-NEDD4 WT or C967S mutant in HEK293T cells. MG132 treatment was carried out as indicated. LATS2 protein levels were quantitated by ImageJ and normalized to β-actin levels. (f) NEDD4ΔN280is able to destabilize LATS2 but not WW45. HA-LATS2 (0.5 μg) and MYC9-WW45 (0.5 μg) were co-transfected with 2 μg of NEDD4WTor NEDD4ΔN280in HEK293T cells. Cell lysates were subjected to immnunoblotting with indicated antibodies. Relative protein levels of WW45 and LATS2 normalized to β-actin are shown (n=3). (g) NEDD4 ubiquitylates LATS2in vivo. HisMax-LATS2, HA-Ubiquitin and FLAG-NEDD4 were co-transfected in HEK293T cells as indicated. Cells were treated with MG132 before harvest. Cell lysates were precipitated with Ni2+-NTA resin and analysed by immunoblotting with indicated antibodies. DMSO, dimethylsulphoxide. Figure 3: LATS kinase is another substrate of NEDD4. ( a ) NEDD4 knockdown enhances staurosporine (STS)-induced apoptosis. HEK293T cells were transfected with NEDD4 siRNA alone or in conjunction with WW45 short hairpin RNA as indicated. At 48 h post transfection, cells were treated with 0.5 μM STS for 12 h before harvest. Cells were then collected for the FACS analysis to determine sub-G1 content or subjected to immunoblotting. WW45 protein levels were quantitated by ImageJ and normalized to β-actin protein levels ( n =3). ( b ) WW45 and LATS2 are stabilized when NEDD4 expression is suppressed. Either scrambled siRNA or si NEDD4 -transfected HEK293T cells were treated with STS (0.5 μM) for 12 h before harvest. Lysates were then analysed by immunoblotting with indicated antibodies. ( c ) WW45 and LATS2, but not MST1, are stabilized by MG132. HEK293T cells were treated with 20 μM MG132 for 4 h as indicated. WW45, MST1 and LATS2 protein levels were quantitated by ImageJ, normalized to β-actin levels and the relative protein levels are shown ( n =4). ( d ) NEDD4 interacts with LATS2 in vivo . HA-LATS2 was transfected with either FLAG-NEDD4 WT or C967S in HEK293T cells as indicated. Cell lysates were immunoprecipitated with anti-FLAG M2 resin and analysed by immunoblotting with indicated antibodies. ( e ) NEDD4 decreases LATS2 protein levels in a dose-dependent manner. HA-LATS2 was co-transfected with either FLAG-NEDD4 WT or C967S mutant in HEK293T cells. MG132 treatment was carried out as indicated. LATS2 protein levels were quantitated by ImageJ and normalized to β-actin levels. ( f ) NEDD4 ΔN280 is able to destabilize LATS2 but not WW45. HA-LATS2 (0.5 μg) and MYC 9 -WW45 (0.5 μg) were co-transfected with 2 μg of NEDD4 WT or NEDD4 ΔN280 in HEK293T cells. Cell lysates were subjected to immnunoblotting with indicated antibodies. Relative protein levels of WW45 and LATS2 normalized to β-actin are shown ( n =3). ( g ) NEDD4 ubiquitylates LATS2 in vivo . HisMax-LATS2, HA-Ubiquitin and FLAG-NEDD4 were co-transfected in HEK293T cells as indicated. Cells were treated with MG132 before harvest. Cell lysates were precipitated with Ni 2+ -NTA resin and analysed by immunoblotting with indicated antibodies. DMSO, dimethylsulphoxide. Full size image MST1 inhibits NEDD4-mediated destabilization of WW45 but not of LATS Given that MST1/2 is involved in the regulation of WW45 stability [7] , [33] , we questioned whether MST1/2 affect NEDD4-mediated WW45 degradation. When MST1 or MST2 was co-expressed, NEDD4-mediated destabilization of WW45 was blocked ( Fig. 4a and Supplementary Fig. 4a ). In addition, WW45 polyubiquitylation by NEDD4 was markedly inhibited by MST1 in a dose-dependent manner ( Fig. 4b ). As the kinase activity of MST1 is dispensable for WW45 stability [7] , [33] , we hypothesized that MST1 physically interrupts the interaction between NEDD4 and WW45. Consistently, along with the protective role of MST1 from the NEDD4-mediated degradation of WW45, there was a clear reduction in the binding proportion of WW45 with NEDD4 ( Fig. 4c ). Of note, no physical interaction was observed between NEDD4 and MST1. It was further validated by co-immunoprecipitation assay of WW45 that the binding degree to MST1 and that of NEDD4 were inversely correlated ( Supplementary Fig. 4b ). These results indicate that MST1 indeed inhibits the interaction between WW45 and NEDD4. Interestingly, MST1 was able to protect WW45 WT only, but not WW45 N198 (which was defective in binding to MST1; Supplementary Fig. 4c ) from NEDD4-mediated degradation ( Supplementary Fig. 4d ). Moreover, neither MST1 ( Fig. 4d ) nor WW45 ( Fig. 4e ) could inhibit NEDD4-mediated LATS2 degradation. 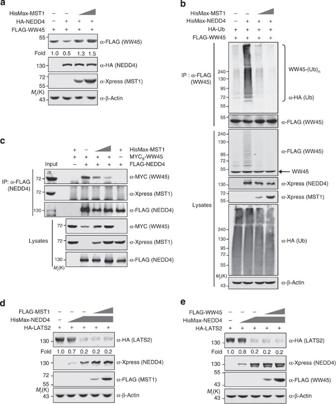Figure 4: MST1 inhibits NEDD4-mediated WW45 downregulation. (a) MST1 interferes with NEDD4 and stabilizes WW45 in a dose-dependent manner. HEK293T cells were transfected with HisMax-MST1, HA-NEDD4 and FLAG-WW45 as indicated. Cell lysates were analysed by immunoblotting with indicated antibodies. WW45 protein levels were quantitated by ImageJ and normalized to β-actin levels. (b) MST1 interferes with NEDD4 and inhibits WW45 ubiquitylation. HEK293T cells were transfected with HisMax-MST1, HisMax-NEDD4, HA-Ubiquitin and FLAG-WW45 as indicated. Cells were treated with 20 μM MG132 for 4 h. Cell lysates were immunoprecipitated with anti-FLAG M2 resin and analysed by immunoblotting with indicated antibodies. (c) MST1 blocks the interaction between WW45 and NEDD4. HisMax-MST1, MYC9-WW45 and FLAG-NEDD4 were transfected into HEK293T cells as indicated. Cell lysates were immunoprecipitated with anti-FLAG M2 resin. NEDD4-bound WW45 or MST1 levels were determined by immunoblotting with indicated antibodies. (d) NEDD4 destabilizes LATS2 in the presence of MST1. HEK293T cells were transfected with HA-LATS2, HisMax-NEDD4 and FLAG-MST1 as indicated. LATS2 protein levels were quantitated by ImageJ and normalized to β-actin levels. (e) NEDD4 destabilizes LATS2 in the presence of WW45. HA-LATS2, HisMax-NEDD4 and FLAG-WW45 were transfected in HEK293T cells as indicated. LATS2 protein levels were quantitated by ImageJ and normalized to β-actin levels. Figure 4: MST1 inhibits NEDD4-mediated WW45 downregulation. ( a ) MST1 interferes with NEDD4 and stabilizes WW45 in a dose-dependent manner. HEK293T cells were transfected with HisMax-MST1, HA-NEDD4 and FLAG-WW45 as indicated. Cell lysates were analysed by immunoblotting with indicated antibodies. WW45 protein levels were quantitated by ImageJ and normalized to β-actin levels. ( b ) MST1 interferes with NEDD4 and inhibits WW45 ubiquitylation. HEK293T cells were transfected with HisMax-MST1, HisMax-NEDD4, HA-Ubiquitin and FLAG-WW45 as indicated. Cells were treated with 20 μM MG132 for 4 h. Cell lysates were immunoprecipitated with anti-FLAG M2 resin and analysed by immunoblotting with indicated antibodies. ( c ) MST1 blocks the interaction between WW45 and NEDD4. HisMax-MST1, MYC 9 -WW45 and FLAG-NEDD4 were transfected into HEK293T cells as indicated. Cell lysates were immunoprecipitated with anti-FLAG M2 resin. NEDD4-bound WW45 or MST1 levels were determined by immunoblotting with indicated antibodies. ( d ) NEDD4 destabilizes LATS2 in the presence of MST1. HEK293T cells were transfected with HA-LATS2, HisMax-NEDD4 and FLAG-MST1 as indicated. LATS2 protein levels were quantitated by ImageJ and normalized to β-actin levels. ( e ) NEDD4 destabilizes LATS2 in the presence of WW45. HA-LATS2, HisMax-NEDD4 and FLAG-WW45 were transfected in HEK293T cells as indicated. LATS2 protein levels were quantitated by ImageJ and normalized to β-actin levels. Full size image NEDD4 retains YAP in the nucleus and increases the YAP transcriptional activity As the activation of the Hippo signalling pathway is reflected by YAP localization, which is critical for YAP activity [13] , [34] , we investigated the effect of NEDD4 on the subcellular localization of YAP using nuclear/cytoplasmic fractionation and immunofluorescence staining. In the absence of Hippo activation signals, YAP shuttles between the cytoplasm and the nucleus [13] , [34] . When the Hippo pathway was activated by ectopic expression of WW45 and LATS2, YAP was found preferentially in the cytoplasm. Such cytoplasmic localization of YAP was further augmented by MST1 co-expression. In contrast, YAP was retained in the nucleus to a significant degree when NEDD4 was co-expressed ( Fig. 5a and Supplementary Fig. 5a ). These results indicate that NEDD4 keeps YAP in the nucleus by inhibiting the Hippo signalling. Because nuclear YAP functions as a transcriptional co-activator, we investigated how NEDD4 affects the expression of YAP downstream target genes using quantitative real-time reverse transcription PCR (RT–PCR) assay. As shown in Fig. 5b , NEDD4 WT but not NEDD4 C967S activated both CTGF (connective tissue growth factor; IGFBP-8 ) and BIRC5 (baculoviral IAP repeat-containing protein-5; apoptosis inhibitor 4; SURVIVIN ) gene expression, both of which are known target genes of YAP [9] , [13] . Next, we tested the effect of NEDD4 on the transcriptional co-activator activity of YAP using the TOPflash luciferase reporter assay [35] . YAP was able to activate the TOPflash but not the FOPflash reporter. LATS2 co-transfection suppressed the TOPflash reporter almost to the basal level, and conversely, additional NEDD4 transfection led to the re-activation of the TOPflash reporter in accordance with the reduction of LATS2 protein ( Fig. 5c ). On the other hand, WW45-binding defective NEDD4 ΔN280 was not able to re-activate the WW45-driven TOPflash reporter, unlike NEDD4 WT . Intriguingly, there was no difference of LATS2-driven TOPflash reporter activity between NEDD4 ΔN280 and NEDD4 WT ( Fig. 5d ), suggesting that NEDD4 may differentially regulate WW45 and LATS2 protein levels. Taken together, NEDD4 modulates the subcellular localization and the transcriptional activity of YAP through the destabilization of WW45 and LATS2. 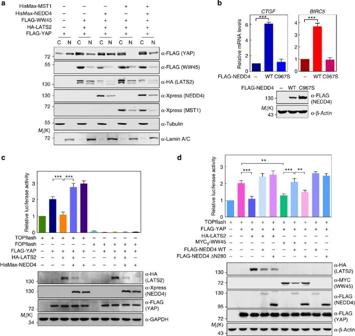Figure 5: NEDD4 controls the YAP localization and activity by regulating WW45 and LATS2. (a) NEDD4 affects the subcellular localization of YAP. FLAG-YAP was co-transfected with FLAG-WW45, HA-LATS2, HisMax-MST1 and HisMax-NEDD4 in HEK293T cells as indicated. Cells were subjected to nuclear cytoplasmic fractionation and analysed by immunoblotting with indicated antibodies. Tubulin and Lamin A/C were used as subcellular localization-specific markers for the cytoplasm and the nucleus, respectively. C, cytoplasmic; N, nuclear fraction. (b) NEDD4 activates YAP-controlled gene expression. Either control vector or FLAG-NEDD4 was transfected in HEK293T cells. Purified total RNA was analysed by quantitative real-time RT–PCR and normalized to the mean values of β-actin and hypoxanthine phosphoribosyltransferse (HPRT). The data are plotted as the mean±s.e.m. of three independent experiments and analysed by one-way analysis of variance (ANOVA) with Bonferroni’s multiple comparison test (***P<0.0001). Corresponding immunoblots are shown below. (c) NEDD4 controls the YAP activity through the regulation of LATS2. HEK293T cells were transfected with following constructs: FLAG-YAP, HA-LATS2, HisMax-NEDD4, β-galactosidase reporter and TOPflash or FOPflash luciferase reporter. The FOPflash reporter plasmid was used as a negative control. Cells were subjected to a luciferase assay or immunoblotting. Luciferase activity was normalized to the β-galactosidase activity. The data are plotted as the mean±s.e.m. of three independent experiments and analysed by one-way ANOVA with Bonferroni’s multiple comparison test (***P<0.0001). (d) NEDD4WTbut not NEDD4ΔN280controls the WW45-driven YAP activity. HEK293T cells were transfected with following constructs: FLAG-YAP, HA-LATS2, MYC9-WW45, FLAG-NEDD4WT, FLAG-NEDD4ΔN280, β-galactosidase reporter and TOPflash or FOPflash luciferase reporter. The FOPflash reporter plasmid was used as a negative control. Cells were subjected to a luciferase assay or immunoblotting. Luciferase activity was normalized to the β-galactosidase activity. The data are plotted as the mean±s.e.m. of three independent experiments and analysed by one-way ANOVA with Bonferroni’s multiple comparison test (**P<0.01, ***P<0.001). Figure 5: NEDD4 controls the YAP localization and activity by regulating WW45 and LATS2. ( a ) NEDD4 affects the subcellular localization of YAP. FLAG-YAP was co-transfected with FLAG-WW45, HA-LATS2, HisMax-MST1 and HisMax-NEDD4 in HEK293T cells as indicated. Cells were subjected to nuclear cytoplasmic fractionation and analysed by immunoblotting with indicated antibodies. Tubulin and Lamin A/C were used as subcellular localization-specific markers for the cytoplasm and the nucleus, respectively. C, cytoplasmic; N, nuclear fraction. ( b ) NEDD4 activates YAP-controlled gene expression. Either control vector or FLAG-NEDD4 was transfected in HEK293T cells. Purified total RNA was analysed by quantitative real-time RT–PCR and normalized to the mean values of β-actin and hypoxanthine phosphoribosyltransferse (HPRT). The data are plotted as the mean±s.e.m. of three independent experiments and analysed by one-way analysis of variance (ANOVA) with Bonferroni’s multiple comparison test (*** P <0.0001). Corresponding immunoblots are shown below. ( c ) NEDD4 controls the YAP activity through the regulation of LATS2. HEK293T cells were transfected with following constructs: FLAG-YAP, HA-LATS2, HisMax-NEDD4, β-galactosidase reporter and TOPflash or FOPflash luciferase reporter. The FOPflash reporter plasmid was used as a negative control. Cells were subjected to a luciferase assay or immunoblotting. Luciferase activity was normalized to the β-galactosidase activity. The data are plotted as the mean±s.e.m. of three independent experiments and analysed by one-way ANOVA with Bonferroni’s multiple comparison test (*** P <0.0001). ( d ) NEDD4 WT but not NEDD4 ΔN280 controls the WW45-driven YAP activity. HEK293T cells were transfected with following constructs: FLAG-YAP, HA-LATS2, MYC 9 -WW45, FLAG-NEDD4 WT , FLAG-NEDD4 ΔN280 , β-galactosidase reporter and TOPflash or FOPflash luciferase reporter. The FOPflash reporter plasmid was used as a negative control. Cells were subjected to a luciferase assay or immunoblotting. Luciferase activity was normalized to the β-galactosidase activity. The data are plotted as the mean±s.e.m. of three independent experiments and analysed by one-way ANOVA with Bonferroni’s multiple comparison test (** P <0.01, *** P <0.001). Full size image NEDD4 controls cell-density-dependent activation of the Hippo pathway It has been established that cell-density-dependent activation of the Hippo pathway leads to YAP phosphorylation followed by inhibition of YAP transcriptional activity [13] . Consistently, YAP was seen in both nucleus and cytoplasm at low cell density but was localized in the cytoplasm when the cells were confluent ( Fig. 6a ). When NEDD4 was suppressed as in NEDD4 KD NIH3T3 stable cells, YAP was localized in the cytoplasm regardless of cell density. It is confirmed by transiently expressed NEDD4 in NIH3T3 cells that co-expression of NEDD4 WT , but not NEDD4 C967S , led to nuclear retention of YAP regardless of cell density ( Supplementary Fig. 6a ). These results indicate that the E3 Ub-ligase activity of NEDD4 is necessary for turning off the cell-density-dependent activation of the Hippo signalling ( Supplementary Fig. 6a ). We also showed that WW45, LATS2 and phosphorylated YAP protein levels were elevated as cell density increased ( Fig. 6b ), confirming that the Hippo pathway was activated when cells reached confluence. Meanwhile, unlike the protein counterparts, mRNA levels of NEDD4, LATS2 and WW45 remained unchanged regardless of the cell density, indicating that WW45 and LATS2 protein levels are post-translationally regulated ( Supplementary Fig. 6b ). It is of note that although NEDD4 acts as a negative regulator of WW45 and LATS2, NEDD4 protein levels were also increased at high cell density ( Fig. 6b ). It is well established that E3 Ub-ligases auto-ubiquitylate to control their own stability [36] , [37] , [38] . This appears to apply to NEDD4 as well. Specifically, we noticed that the protein level of the E3 Ub-ligase-defective NEDD4 C967S mutant was always higher than that of NEDD4 WT ( Figs 2b and 3d ), indicating that the stability of NEDD4 itself might be regulated by auto-ubiquitylation. Thus, we speculated that the elevation of NEDD4 protein levels at high cell density (shown in Fig. 6b ) was due to a reduction in the E3 Ub-ligase activity of NEDD4. To address this hypothesis, we analysed the E3 Ub-ligase activity and stability of NEDD4 at low and high cell densities. Auto-ubiquitylation of NEDD4 at high cell density was declined drastically compared with that at low cell density ( Supplementary Fig. 6c ). Consistently, NEDD4 at high cell density was more stable than NEDD4 at low cell density, providing a basis for the increase in protein levels and activation of the Hippo pathway components ( Supplementary Fig. 6d ). Next, we examined the dependency of WW45 and LATS2 protein levels on NEDD4 using NEDD4 KD NIH3T3 stable cells. When NEDD4 was scarce, protein levels of WW45 and LATS2 were constantly high regardless of cell density ( Fig. 6c ) and their ubiquitylation was barely detected ( Supplementary Fig. 6e ). However, their specific interaction was not altered as cell density changed ( Supplementary Fig. 6f ). These data suggest that the stabilization of WW45 and LATS2 at high cell density is mainly dependent on NEDD4 activity. YAP was phosphorylated even at low cell density in NEDD4 KD cells ( Fig. 6c ), indicating that elevated protein levels of WW45 and LATS2 by NEDD4 depletion lead to YAP phosphorylation. Moreover, quantitative real-time RT–PCR analyses revealed that YAP transcriptional activity was also dependent on NEDD4. Expression levels of YAP target genes, Ctgf , Birc5 , Inhba (Inhibin beta A chain) and Mcl1 (induced myeloid leukemia cell differentiation protein Mcl-1 homologue; Bcl-2-related protein EAT/mcl1) [9] , [13] , were decreased at high cell density in NIH3T3 control cells but remained low in NEDD4 KD cells regardless of cell density ( Fig. 6d and Supplementary Fig. 6g ). Furthermore, NEDD4 KD cells grew slower than control cells and this growth suppression was partially recovered by combined double KD of either WW45 or LATS2 in NEDD4 KD cells ( Figs 6e,f ). Taken together, our results demonstrate that cell-density-dependent activation of the Hippo pathway is due to the changes of NEDD4 E3 Ub-ligase activity. In addition, NEDD4 depletion leads to the activation of the Hippo pathway accompanied by reduced proliferation. 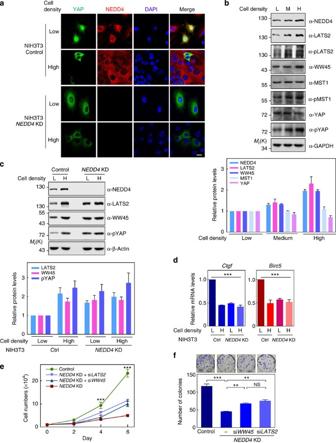Figure 6: NEDD4 is involved in the cell-density-dependent activation of the Hippo pathway. (a) NEDD4 modulates the density-dependent subcellular localization of YAP. GFP-YAP was transfected in NIH3T3 control cells or NIH3T3-NEDD4KD cells. At 24 h post transfection, cells were cultured as either sparse subconfluent or dense confluent monolayers. Cells were subjected to immunofluorescence staining and the subcellular localization of YAP and NEDD4 was visualized under a LSM710 multi-photon confocal laser scanning microscope (Zeiss). The scale bar represents 10 μm. (b) Cell density affects the protein levels of the Hippo pathway components as well as NEDD4. Equal numbers of NIH3T3 cells (1.3 × 105) were seeded in a different size of culture dishes to achieve the different cell density (L, low cell density to 100 mm dish; M, medium cell density to 60 mm dish; H, high cell density to 35 mm dish). After 24 h incubation, cells were subjected to immunoblotting. Relative protein levels quantitated by ImageJ and normalized to glyceraldehyde 3-phosphate dehydrogenase (GAPDH) are shown (n=3). (c) WW45 and LATS2 protein levels remain unchanged regardless of cell density inNEDD4KD stable cells. Control orNEDD4KD NIH3T3 cells were cultured sparsely or to maximum confluence for 24 h and then subjected to immunoblotting. Relative protein levels quantitated by ImageJ and normalized to β-actin are shown (n=3). (d) Expression of YAP-controlled genes is inhibited inNEDD4KD cells. Total RNA isolated from either control orNEDD4KD stable NIH3T3 cells was used for quantitative real-time RT–PCR analyses. Normalization was carried out with respect to the mean values of β-actin and hypoxanthine phosphoribosyltransferse (HPRT). Data are plotted as the mean±s.e.m. of five independent experiments and analysed by one-way analysis of variance (ANOVA) with Bonferroni’s multiple comparison test (***P<0.0001). (e,f) Growth suppression ofNEDD4KD cells was partially recovered by simultaneous knockdown with either siWW45or siLATS2inNEDD4KD cells. (e) Control orNEDD4KD stable cells were transfected with indicated siRNAs and replated for the subsequent proliferation assay. Data are plotted as the mean±s.e.m. of four independent experiments and analysed by one-way ANOVA with Bonferroni’s multiple comparison test (***P<0.0001). (f) Control orNEDD4KD stable cells were transfected with indicated siRNAs. At 24 h post transfection, 150 cells were seeded into six-well plates and formed colonies were scored after 10 days. Data are plotted as the mean±s.e.m. of three independent experiments and representative plates are shown. DAPI, 4',6-diamidino-2-phenylindole. Figure 6: NEDD4 is involved in the cell-density-dependent activation of the Hippo pathway. ( a ) NEDD4 modulates the density-dependent subcellular localization of YAP. GFP-YAP was transfected in NIH3T3 control cells or NIH3T3- NEDD4 KD cells. At 24 h post transfection, cells were cultured as either sparse subconfluent or dense confluent monolayers. Cells were subjected to immunofluorescence staining and the subcellular localization of YAP and NEDD4 was visualized under a LSM710 multi-photon confocal laser scanning microscope (Zeiss). The scale bar represents 10 μm. ( b ) Cell density affects the protein levels of the Hippo pathway components as well as NEDD4. Equal numbers of NIH3T3 cells (1.3 × 10 5 ) were seeded in a different size of culture dishes to achieve the different cell density (L, low cell density to 100 mm dish; M, medium cell density to 60 mm dish; H, high cell density to 35 mm dish). After 24 h incubation, cells were subjected to immunoblotting. Relative protein levels quantitated by ImageJ and normalized to glyceraldehyde 3-phosphate dehydrogenase (GAPDH) are shown ( n =3). ( c ) WW45 and LATS2 protein levels remain unchanged regardless of cell density in NEDD4 KD stable cells. Control or NEDD4 KD NIH3T3 cells were cultured sparsely or to maximum confluence for 24 h and then subjected to immunoblotting. Relative protein levels quantitated by ImageJ and normalized to β-actin are shown ( n =3). ( d ) Expression of YAP-controlled genes is inhibited in NEDD4 KD cells. Total RNA isolated from either control or NEDD4 KD stable NIH3T3 cells was used for quantitative real-time RT–PCR analyses. Normalization was carried out with respect to the mean values of β-actin and hypoxanthine phosphoribosyltransferse (HPRT). Data are plotted as the mean±s.e.m. of five independent experiments and analysed by one-way analysis of variance (ANOVA) with Bonferroni’s multiple comparison test (*** P <0.0001). ( e , f ) Growth suppression of NEDD4 KD cells was partially recovered by simultaneous knockdown with either si WW45 or si LATS2 in NEDD4 KD cells. ( e ) Control or NEDD4 KD stable cells were transfected with indicated siRNAs and replated for the subsequent proliferation assay. Data are plotted as the mean±s.e.m. of four independent experiments and analysed by one-way ANOVA with Bonferroni’s multiple comparison test (*** P <0.0001). ( f ) Control or NEDD4 KD stable cells were transfected with indicated siRNAs. At 24 h post transfection, 150 cells were seeded into six-well plates and formed colonies were scored after 10 days. Data are plotted as the mean±s.e.m. of three independent experiments and representative plates are shown. DAPI, 4',6-diamidino-2-phenylindole. Full size image NEDD4 acts as an essential regulator of the Hippo/Yorkie pathway in Drosophila The Hippo signalling pathway was originally discovered in Drosophila and is highly conserved from flies to humans [1] , [2] , [6] , [10] , [21] . However, it is still unknown whether Drosophila Nedd4, the homologue of human NEDD4, functions in the Hippo pathway. Therefore, we sought to confirm and characterize the novel functions of Nedd4 as an essential modulator for the Hippo pathway using the genetically amenable Drosophila model organism. For this, we examined expression levels of expanded ( ex ), a well-known target of Hippo signalling, by using ex-lacZ reporter in wing imaginal discs with Nedd4 mutant clones. The result showed that ex-lacZ expression was diminished in Nedd4 mutant cells when compared with adjacent wild-type cells ( Fig. 7a ). These data demonstrate that Nedd4 acts as a regulator of Hippo pathway in wing imaginal disc. 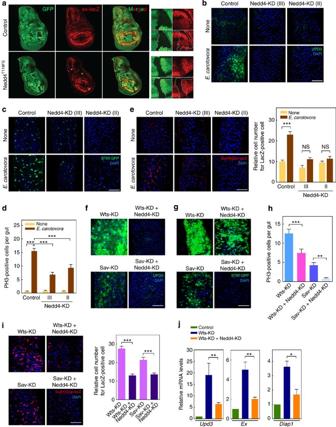Figure 7: NEDD4 genetically interacts with the Hippo pathway inDrosophila. The specific genotypes of fly lines used in this study are described in theSupplementary Table 1. (a) Nedd4 is required for optimal Yki-target gene expression in wing imaginal discs. Arrowheads indicate that GFP-negativeNedd4mutant clones showed reduced ex-LacZ expression when compared with adjacent GFP-positive wild-type cells. Regions in dotted boxes in control and Nedd4T119FSdiscs were magnified and shown. In this region, GFP (green) and ex-LacZ (red) expression were shown with or without clone borders. (b) Nedd4 is required for infection-induced Yki-targetUpd3expression in adult enterocytes.Upd3-GAL3>UAS-GFPexpression (at 4 h post-bacterial infection) was monitored in the presence or absence ofNedd4-KD. (c–e) Nedd4 is involved in the Hippo pathway-controlled epithelial cell renewal process following pathogen infection. Enterocyte-specificNedd4-KD flies usingMyo1A-GAL4were used in this study. JAK-STAT activation level (c), ISC proliferation (d) and differentiation rate (e) were analysed by monitoring STAT-dependent GFP reporter (STAT-GFP), PH3-positive cells and aSu(H)Gbe-lacZ-positive EB, respectively. STAT reporter analysis and ISC proliferation/differentiation were examined at 4 and 16 h post-bacterial infection, respectively. EB cells in midguts were analysed with anti-LacZ antibodies. Nuclear staining was performed with 4',6-diamidino-2-phenylindole (DAPI). For the quantitative analysis of EB cells, the relative number of LacZ-positive cells was determined by counting the number of LacZ-positive cells per 100 DAPI-positive cells in multiple images. Data indandewere analysed using an analysis of variance (ANOVA) followed by Tukey and Tamhane’s T2 test, respectively; values represent mean±s.e.m. (***P<0.001) of at least three independent experiments. NS denotes not significant. The scale bar represents 100 μm. (f–i) The high levels of Upd3-JAK-STAT activity and epithelial cell renewal rate upon the suppression of Hippo signalling were greatly attenuated by boosting the Hippo pathway activity throughNedd4-KD.Upd3-GAL3>UAS-GFPexpression (at 4 h post-bacterial infection) was monitored (f). Enterocyte-specific KD flies usingMyo1A-GAL4were used to analyse STAT activity (g), PH3-positive ISC (h) and aSu(H)Gbe-lacZ-positive EB (i). Data inhandiwere analysed using an ANOVA followed by Tukeypost hoctest; values represent mean±s.e.m. (**P<0.005, ***P<0.001) of at least three independent experiments. The scale bar represents 100 μm. (j) Analysis of Hippo target gene expression inNedd4-KD animals.Upd3, exandDiap1expression were analysed using midgut by quantitative PCR analysis. Target gene expression in the control flies (w1118) was taken arbitrarily as 1. Conditional gene KD in the enterocytes was performed by usingMyo1Ats–GAL4(combiningMyo1A-GAL4and a temperature sensitive GAL4 inhibitor,tub-GAL80ts). To temporarily control targetRNAiexpression by usingMyo1Ats–GAL4, flies (maintained at 18 °C) were shifted to 29 °C for 5 days to initiate the targetRNAiexpression. Relative expression levels are expressed as the mean±s.e.m. of at least three independent experiments (*P<0.05, **P<0.005). Figure 7: NEDD4 genetically interacts with the Hippo pathway in Drosophila . The specific genotypes of fly lines used in this study are described in the Supplementary Table 1 . ( a ) Nedd4 is required for optimal Yki-target gene expression in wing imaginal discs. Arrowheads indicate that GFP-negative Nedd4 mutant clones showed reduced ex-LacZ expression when compared with adjacent GFP-positive wild-type cells. Regions in dotted boxes in control and Nedd4 T119FS discs were magnified and shown. In this region, GFP (green) and ex-LacZ (red) expression were shown with or without clone borders. ( b ) Nedd4 is required for infection-induced Yki-target Upd3 expression in adult enterocytes. Upd3-GAL3>UAS-GFP expression (at 4 h post-bacterial infection) was monitored in the presence or absence of Nedd4 -KD. ( c – e ) Nedd4 is involved in the Hippo pathway-controlled epithelial cell renewal process following pathogen infection. Enterocyte-specific Nedd4 -KD flies using Myo1A-GAL4 were used in this study. JAK-STAT activation level ( c ), ISC proliferation ( d ) and differentiation rate ( e ) were analysed by monitoring STAT-dependent GFP reporter (STAT-GFP), PH3-positive cells and a Su(H)Gbe-lacZ -positive EB, respectively. STAT reporter analysis and ISC proliferation/differentiation were examined at 4 and 16 h post-bacterial infection, respectively. EB cells in midguts were analysed with anti-LacZ antibodies. Nuclear staining was performed with 4',6-diamidino-2-phenylindole (DAPI). For the quantitative analysis of EB cells, the relative number of LacZ-positive cells was determined by counting the number of LacZ-positive cells per 100 DAPI-positive cells in multiple images. Data in d and e were analysed using an analysis of variance (ANOVA) followed by Tukey and Tamhane’s T2 test, respectively; values represent mean±s.e.m. (*** P <0.001) of at least three independent experiments. NS denotes not significant. The scale bar represents 100 μm. ( f – i ) The high levels of Upd3-JAK-STAT activity and epithelial cell renewal rate upon the suppression of Hippo signalling were greatly attenuated by boosting the Hippo pathway activity through Nedd4 -KD. Upd3-GAL3>UAS-GFP expression (at 4 h post-bacterial infection) was monitored ( f ). Enterocyte-specific KD flies using Myo1A-GAL4 were used to analyse STAT activity ( g ), PH3-positive ISC ( h ) and a Su(H)Gbe-lacZ -positive EB ( i ). Data in h and i were analysed using an ANOVA followed by Tukey post hoc test; values represent mean±s.e.m. (** P <0.005, *** P <0.001) of at least three independent experiments. The scale bar represents 100 μm. ( j ) Analysis of Hippo target gene expression in Nedd4 -KD animals. Upd3, ex and Diap1 expression were analysed using midgut by quantitative PCR analysis. Target gene expression in the control flies ( w 1118 ) was taken arbitrarily as 1. Conditional gene KD in the enterocytes was performed by using Myo1A ts –GAL4 (combining Myo1A-GAL4 and a temperature sensitive GAL4 inhibitor, tub-GAL80 ts ). To temporarily control target RNAi expression by using Myo1A ts –GAL4 , flies (maintained at 18 °C) were shifted to 29 °C for 5 days to initiate the target RNAi expression. Relative expression levels are expressed as the mean±s.e.m. of at least three independent experiments (* P <0.05, ** P <0.005). Full size image In Drosophila , it has recently been reported that the Hippo pathway is rapidly inactivated in intestinal enterocytes (ECs) in response to tissue injury, leading to the activation of transcriptional co-activator Yki [21] , [22] , [39] , [40] . Activated Yki is known to induce the expression of cytokine Unpaired-3 ( Upd3 ) in ECs that in turn activates JAK-signal transducers and activators of transcription (STAT) signalling pathway in progenitor cells such as enteroblasts (EBs) and ISCs [21] , [22] , [39] , [41] . It has been shown that Hippo pathway inactivation in EC and subsequent JAK-STAT pathway activation in progenitor cells are of central importance for the epithelial renewal process (that is, ISC proliferation and differentiation into EB and EC) to replenish the damaged EC [21] , [22] . To investigate whether Nedd4 in EC is involved in epithelial cell renewal process via regulating the Hippo pathway, we examined infection-induced Upd3 expression in EC in a Nedd4-KD condition. When we introduced the expression of Nedd4-RNAi , we found that infection-induced Upd3 expression was greatly reduced ( Fig. 7b ), indicating that Nedd4 regulates the Hippo pathway in ECs. Two independent Nedd4-RNAi lines showed similar results. Furthermore, the infection-induced JAK-STAT activation (by monitoring STAT-dependent green fluorescent protein (GFP) reporter) in progenitor cells and augmented ISC proliferation/differentiation rate (by monitoring number of dividing cells using an anti-phosphorylated histone 3 (PH3) antibody and Su(H)Gbe-lacZ -positive EB accumulation) found in wild-type flies were almost completely abolished in animals carrying EC-specific Nedd4 -KD ( Fig. 7c–e ). These results indicate that Nedd4-mediated Hippo pathway inactivation and subsequent Upd3 induction in ECs are required for epithelial cell renewal process following pathogen infection. Consistent with this notion, inactivation of Hippo pathway in EC, by using Wts -KD or Sav -KD, is sufficient to induce all events necessary for epithelial cell renewals (that is, Upd3 induction in ECs, STAT-GFP reporter activation in progenitor cells, ISC proliferation and EB accumulation) even in the absence of pathogen infection ( Fig. 7f–i ). Importantly, the high epithelial cell renewal rate induced by downregulating the Hippo pathway activity in EC was greatly attenuated by boosting the Hippo pathway activity through Nedd4 -KD in EC ( Fig. 7f–i ). Consistent with Hippo-modulated Upd3 expression, high expression levels of different Hippo target genes such as DIAP1 and ex were also found in flies with reduced Hippo pathway activity (that is, Wts -KD flies), and this high expression level could be significantly diminished by enhancing the Hippo pathway activity (that is, Wts/Nedd4 double KD; Fig. 7j ). As reduced Wts protein level in the intestine of Wts -KD animal can be augmented in Wts/Nedd4 double KD animals ( Supplementary Fig. 7a ), the suppression of the high epithelial cell renewal rates of flies with reduced Hippo pathway activity by Nedd4 -KD is most likely due to a reciprocal compensatory effect of the two opposing KD phenotypes (for example, Hippo pathway downregulation by Wts -KD versus Hippo pathway upregulation by Nedd4 -KD). Taken together, these results demonstrate that Nedd4 genetically interacts with the Hippo pathway, and that Nedd4 acts as an essential signalling component in the Hippo pathway in gut cell homeostasis. In the present study, we have identified NEDD4 as a new regulatory component of the Hippo signalling pathway. Our results show that NEDD4 plays a crucial role in regulating cell proliferation and apoptosis in both mammalian cells and Drosophila . NEDD4 depletion leads to escalated apoptosis and reduced proliferation, which are typical outcomes of the activated Hippo pathway. Accordingly, NEDD4 negatively regulates core components of the Hippo pathway, WW45 and LATS1/2. Both proteins are polyubiquitylated by NEDD4 and subsequently degraded by the 26S proteasome, leading to inactivation of the Hippo pathway. Given that NEDD4 negatively regulates the stability of WW45 and that MST1 interferes with this destabilization, a new underlying mechanism of WW45 stabilization by MST1/2 can be speculated. We have shown that MST1/2 inhibits WW45 ubiquitylation by hindering its interaction with NEDD4 and the binding degree of MST1 to WW45 was greatly increased not only in the overexpressed conditions but also in the confluent culture conditions, which indicates that WW45 protein levels are regulated by a fine balance between NEDD4 and MST1. As the binding regions of WW45 to MST1 and to NEDD4 are different, a direct binding competition between them is not likely, as seen in the case of RASSF6 and MST2 (ref. 42 ). Although overall MST1 protein levels were not changed by cell density, phosphorylated MST1, which is associated with its activity, was increased at high cell density, therefore, it is plausible that MST1 becomes more active and predominantly interacts with WW45 at high cell density. Meanwhile, NEDD4 becomes inactive, which was monitored by autoubiquitylation and substrate ubiquitylation, but its interaction to WW45 remains unchanged at high cell density. Thus, it is most likely that the shifted binding preference of WW45 from NEDD4 to MST1 at high cell density may contribute to determine the WW45 protein levels. On the other hand, high levels of either WW45 or MST1 were not able to protect LATS1/2 against NEDD4, which is consistent with previous findings that Warts protein levels can be regulated by alternative mechanism independent of Salvador and Hippo in Drosophila [34] , [43] . KIBRA was recently identified as a component of the mammalian Hippo signalling [44] in addition to genetic studies in Drosophila [45] , [46] , [47] . Similar to NEDD4, the WW domain of KIBRA is necessary for binding to LATS2 and KIBRA thus stabilizes and activates LATS2 by inhibiting ubiquitylation. Although how KIBRA is involved in the NEDD4-mediated LATS2 regulation remains to be elucidated, it is possible that KIBRA and NEDD4 compete with each other for LATS2. It has also been reported that LATS1 is regulated by ITCH, an E3 Ub-ligase that belongs to the NEDD4 family [29] , [30] . Thus, we sought to further delineate the specificity of NEDD4 on regulating the Hippo pathway. N-terminal amino-acid sequence alignment of NEDD4 family member proteins [48] , including NEDD4, NEDD4L (also known as NEDD4-2), ITCH, WWP1 and WWP2, showed that only NEDD4 has specific N-terminal 100-amino-acid region, which is critical for binding to WW45 compared with other family members ( Supplementary Fig. 1b ). On the other hand, ITCH can interact with LATS1, but not with either WW45 or LATS2 ( Supplementary Fig. 1c–e ), followed by LATS1 destabilization. It has recently been reported that LATS1 stability can be controlled by NEDD4 (ref. 31 ). Therefore, it would be possible that NEDD4 and ITCH regulate LATS1 together or independently of the other depending on physiological or cellular context and NEDD4 could function as the E3 Ub-ligase for both LATS1 and LATS2. Activation of the Hippo pathway is manifested by the activation of LATS whose stabilization and phosphorylation are both required [34] , [43] . As elevated LATS protein levels are able to act on YAP even without its phosphorylation [9] , [13] , it is very important to maintain LATS protein levels precisely. In this regard, it is worthy of note that NEDD4 is able to control LATS activation directly through the negative regulation of LATS stability and indirectly through the negative regulation of WW45, which is essential for the core signalling cascade of WW45-MST-mediated LATS phosphorylation. Thus, NEDD4 is able to block the activation of LATS efficiently and thereby tightly regulates the Hippo signalling pathway ( Fig. 8 ; see the corresponding legend for further details). 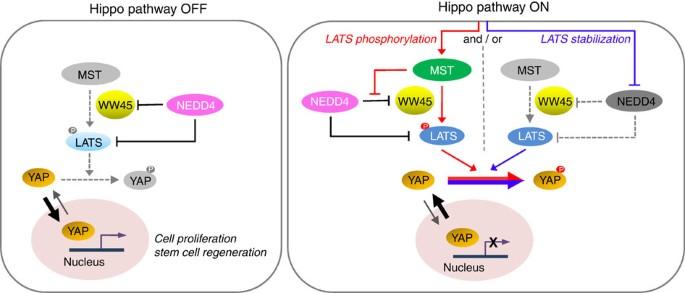Figure 8: A proposed model for NEDD4 on regulating the Hippo signalling pathway. NEDD4 tightly regulates the Hippo pathway through WW45 and LATS destabilization. WW45 and LATS protein levels are maintained low by NEDD4-mediated degradation, which confers Hippo OFF state. YAP dominantly enters nuclei and induces its target gene expression by interacting with transcription factors, promoting cell proliferation or intestinal stem cell renewal. When cells receive the Hippo activation signalling (that is, ‘LATS phosphorylation’ and/or ‘LATS stabilization’), YAP is phosphorylated by LATS and subsequently sequestered in the cytoplasm. ‘LATS phosphorylation’ signal activates MST, and activated MST stabilizes WW45 by inhibiting NEDD4-mediated degradation. MST then phosphorylates LATS with WW45. On the other hand, ‘LATS stabilization’ signal inhibits NEDD4 activity, which leads to the elevated LATS as well as WW45 protein levels. As LATS activity is controlled dually by its phosphorylation and stabilization34,43, kinase-relayed phosphorylation signals and stabilization signals work in concert to fully activate LATS to its maximum extent followed by Hippo ON state. Figure 8: A proposed model for NEDD4 on regulating the Hippo signalling pathway. NEDD4 tightly regulates the Hippo pathway through WW45 and LATS destabilization. WW45 and LATS protein levels are maintained low by NEDD4-mediated degradation, which confers Hippo OFF state. YAP dominantly enters nuclei and induces its target gene expression by interacting with transcription factors, promoting cell proliferation or intestinal stem cell renewal. When cells receive the Hippo activation signalling (that is, ‘LATS phosphorylation’ and/or ‘LATS stabilization’), YAP is phosphorylated by LATS and subsequently sequestered in the cytoplasm. ‘LATS phosphorylation’ signal activates MST, and activated MST stabilizes WW45 by inhibiting NEDD4-mediated degradation. MST then phosphorylates LATS with WW45. On the other hand, ‘LATS stabilization’ signal inhibits NEDD4 activity, which leads to the elevated LATS as well as WW45 protein levels. As LATS activity is controlled dually by its phosphorylation and stabilization [34] , [43] , kinase-relayed phosphorylation signals and stabilization signals work in concert to fully activate LATS to its maximum extent followed by Hippo ON state. Full size image It has been reported that environmental cues (for example, cell density) determine the activation of the Hippo pathway [13] , [49] . When cells in culture reach confluence, the Hippo pathway is activated, thus ensuing phosphorylation and inactivation of YAP ultimately induce contact inhibition [13] . We also observed that phosphorylation and subcellular localization of YAP are indeed modulated by changes in cell density. In addition, it has been reported that WW45- and LATS2-KO mouse embryonic fibroblast cells lose contact inhibition, similar to cancer cells [50] , [51] . However, it is still largely unknown how the Hippo pathway becomes active as cell density increases. As shown in the present study, NEDD4 Ub-ligase activity seems essential for Hippo signalling in this regard as well. At low cell density, NEDD4 inhibits the activation of the Hippo pathway by maintaining WW45 and LATS proteins at low levels. NEDD4 becomes inactive at high cell density, resulting in the stabilization of WW45 and LATS followed by subsequent activation of the Hippo pathway. One of the intriguing observations presented here is that NEDD4 activity is altered by changes in cell density. NEDD4 becomes stabilized at high cell density. NEDD4 is known to be auto-inhibited by intramolecular interaction between C2 and HECT domains [37] , and calcium influx into cells releases C2 domain from HECT domain thereby activating the E3 Ub-ligase activity of NEDD4 (ref. 27 ). As epidermal growth factor receptor (EGFR) and/or acetylcholine receptor signalling pathways are able to elevate intracellular calcium levels and then activate NEDD4 (ref. 27 ), it would be of interest to test whether the Hippo pathway is in turn regulated by EGFR and/or acetylcholine receptor signalling via the activation of NEDD4. Moreover, NEDD4 WT is able to block the accumulation of cytoplasmic YAP even at high cell density, whereas the catalytically inactive NEDD4 C967S mutant fails to do so. NEDD4 is known to promote cell growth as an oncoprotein and NEDD4 KO mouse shows severe growth retardation [28] . Consistently, NEDD4 KD cells show slower cell proliferation and higher apoptosis, indicating that the Hippo pathway is abnormally activated by the dysregulation of WW45 and LATS. Importantly, simultaneous double KD of NEDD4 with WW45 or LATS2 partially restores cell growth or reduces apoptosis in part. Taken together, these data indicate that NEDD4 positively controls cell proliferation through the negative regulation of WW45 and LATS. This would in turn imply that NEDD4 affects cell growth and tumorigenesis via Hippo signalling. The NEDD4-regulated Hippo signalling cascade is further validated in Drosophila . Our study suggests that infection-induced Nedd4 activation leads to the inactivation of the Hippo pathway and subsequent Upd3 expression in ECs that in turn activates the JAK-STAT pathway for the transition from ISC to EB and EC. Nedd4 -KD animals having defects in epithelial cell renewal showed severe mortality to gut infection ( Supplementary Fig. 7b ), and this high mortality could be significantly ameliorated by enhancing the Hippo pathway activity (that is, double KD flies for Sav-RNAi plus Nedd4-RNAi ) or by re-introducing Nedd4 ( Supplementary Fig. 7b ). In addition to the involvement of Nedd4 in epithelial cell renewal in the gut, we found that Nedd4 is also involved in gut size determination via regulating the Hippo pathway ( Supplementary Fig. 7c ). Furthermore, Nedd4 -KD is sufficient to decrease adult wing sizes ( Supplementary Fig. 7d ). All of these observations indicate that Nedd4 acts as an essential signalling component in gut cell homeostasis and host survival during gut–pathogen interactions by modulating the Hippo pathway activity. Overall, our study defines a previously unknown level of control in the Hippo signalling and sheds a new light on the regulatory mechanism of the Hippo pathway establishing NEDD4 as an essential signalling component of the pathway. Cell culture and fly strains NIH3T3 and HEK293T cells were maintained in DMEM supplemented with 100 U ml −1 of penicillin, 100 μg ml −1 of streptomycin and 10% fetal bovine serum (Gibco) at 37 °C in a humidified 5% CO 2 atmosphere. Transient transfection was carried out using either polyethylenimine (Sigma) or Lipofectamine 2000 (Invitrogen) according to the manufacturer’s instructions. Nuclear and cytoplasmic fractionations were performed using Nuclear Extract Kit (Active Motif). The fly lines used in this study were: w 1118 , esg-GAL4>UAS-GFP [52] ; Upd3-GAL4>UAS-GFP [53] ; Su(H)Gbe-LacZ [54] ; Myo1A-GAL4 (ref. 55 ); Nedd4 T119FS (ref. 56 ); ex-lacZ [57] and tub-GAL80 ts (ref. 55 ). A transgenic fly carrying 10XSTAT-GFP was used to monitor JAK-STAT pathway activity [58] . RNAi lines for Wts , Sav and Nedd4 were obtained from Vienna Drosophila RNAi Center. Two independent Nedd4-KD lines, Nedd4 (II) and Nedd4 (III), correspond to VDRC #108475 and #13121, respectively, were obtained. The genotypes of fly lines used in this study were as described in Supplementary Table 1 . Immunoblotting and antibodies Immunoblotting was performed using standard protocol. Rabbit polyclonal anti-WW45 antiserum was raised against a recombinant GST-WW45. Anti-Wts antibody (kind gift from Dr K. D. Irvine, Rutgers University) was used as described previously [23] . Other antibodies were used as follows: anti-NEDD4 and anti-ITCH (BD Biosciences); anti-FLAG and anti-β-actin (1:5,000 dilution; Sigma); anti-ubiquitin, anti-PARP, anti-Lamin A/C, anti-YAP, anti-MYC and anti-HA (Santa Cruz Biotechnology); anti-Xpress (1:5,000 dilution; Invitrogen); anti-glyceraldehyde 3-phosphate dehydrogenase, anti-pYAP, anti-pLATS1/2, anti-pMST1 and anti-MST1 (Cell Signaling Technology); anti-LATS2 (Bethyl Laboratories Inc.); anti-Tubulin (Chemicon); peroxidase-conjugated AffiniPure goat anti-rabbit and anti-mouse IgGs (Bio-Rad). Antibody dilution for immunoblotting is 1:1,000, unless indicated otherwise. Uncropped full scanned immunoblots can be found in Supplementary Fig. 9 . Relative protein levels in the main immunoblot figures were quantitated by ImageJ and normalized to either β-actin or glyceraldehyde 3-phosphate dehydrogenase levels. Values are plotted as the mean±s.e.m. of at least three independent experiments. RNA interference Cells were transfected with Lipofectamine 2000 reagent (Invitrogen) according to the manufacturer’s protocol. The following sequences were used: si NEDD4 #1, sense, 5′- CGAAGAUCACCUCUCUUACdTdT -3′, antisense, 3′- dTdTGCUUCUAGUGGAGAGAAUG -5′; si NEDD4 #2, sense, 5′- UUAGAGCCUGGCUGGGUUGdTdT -3′, antisense, 3′- dTdTAAUCUCGGACCGACCCAAC -5′; si NEDD4 #3, sense, 5′- UCCAAAGUGGAAUGAAGAAdTdT -3′, antisense, 3′- dTdTAGGUUUCACCUUACUUCUU -5′; si ITCH , sense, 5′- CGGGCGAGUUUACUAUGUAdTdT -3′, antisense, 3′- dTdTGCCCGCUCAAAUGAUACAU -5′. For KD of WW45, the targeted WW45 oligonucleotide primer (sh WW45 #1, 5′- CCATGATCTCTTCCAAAGA -3′; sh WW45 #2, 5′- GAATTTGGAACCTATTA -3′) was designed and inserted in the pSilencer 2.0-U6 plasmid vector (Ambion). siRNAs were synthesized by Samchully Pharm or otherwise purchased from Santa Cruz Biotechnology. Immunoprecipitation Cells were collected in a lysis buffer (20 mM Tris-HCl (pH 7.5), 150 mM NaCl, 0.2% Triton X-100) supplemented with 1 × complete protease inhibitor cocktail (Roche) and incubated with anti-FLAG M2 resin (Sigma) for 2 h at 4 °C. Immunoprecipitated resin was washed three times with TNET buffer (20 mM Tris-HCl (pH 7.5), 150 mM NaCl, 0.1 mM EDTA and 0.2% Triton X-100) and two times with TNE buffer (20 mM Tris-HCl (pH 7.5), 150 mM NaCl and 0.1 mM EDTA). Bound proteins were eluted, resolved by SDS–polyacrylamide gel electrophoresis, and analysed by either coomassie staining or immunoblotting with indicated antibodies. Assays for ubiquitylation and pulse-chase analysis For the in vitro ubiquitylation assay, purified GST-WW45 or His-LATS2 (0.8 μg) from E. coli was incubated at 37 °C for 2 h with E1 (1 μg), Ubc5 (2 μg) and Ub (10 μg), ATP-regenerating system (50 mM Tris-HCl (pH 7.5), 5 mM MgCl 2 , 10 mM creatine phosphate, 5 U ml −1 of phosphocreatine kinase and 5 mM ATP) and 1 × complete protease inhibitor cocktail in the presence or absence of NEDD4 (1 μg) purified from HEK293T cells. After incubation, each sample was subjected to SDS–polyacrylamide gel electrophoresis and immunoblotting with anti-WW45 or anti-LATS2 antibody. For the pulse-chase analysis, transfected HEK293T cells were treated with CHX (200 μg ml −1 ) for indicated times. Cell lysates were subjected to immunoblotting with appropriate antibodies. Flow cytometry HEK293T cells were transfected with appropriate siRNAs including scrambled control and treated with STS. Cells were collected, washed with PBS and fixed with 70% ethanol. Fixed cells were permeabilized by 0.3% Triton X-100 and stained in propidium iodide solution containing RNase A (250 μg ml −1 ). Propidium iodide-stained cells were then analysed for their DNA content using a fluorescence-activated cell sorting instrument (BD Biosciences). Immunofluorescence staining Cells on gelatin-coated coverslips were fixed with 2% formaldehyde in PBS for 30 min at room temperature and permeabilized with 0.5% Triton X-100 in PBS. All subsequent dilutions and washes were performed with PBS containing 0.1% Triton X-100 (PBS-T). Nonspecific binding sites were masked by incubation for 30 min with blocking solution consisting of 10% goat serum, 1% BSA and 1% gelatin in PBS. Cells were incubated with primary antibody for 1 h, washed four times with PBS-T for 10 min each, and then incubated with either Alexa Fluor 488- or Alexa Fluor 555-conjugated secondary antibody for 1 h. The coverslips were washed four times and mounted using Vectashield (Vector Labs). 4',6-Diamidino-2-phenylindole was used to counterstain the nuclei. Cells were visualized under a LSM710 multi-photon confocal laser scanning microscope (Zeiss). Clonal analysis Clonal analysis was performed by using the FLP/FRT system [59] . The animals (24–72 h after egg laying) were subjected to 37 °C for 60 min to induce FLP recombinase. Animals were dissected at the third instar larval stage. Real-time RT–PCR Total RNA was isolated from cells using the easy-BLUE total RNA extraction kit (iNtRON Biotechnology). Reverse transcription reactions were performed using RevertAid M-MuLV reverse transcriptase (Fermentas) and oligo (dT) primer according to the manufacturer’s instructions. Real-time PCR was performed using a KAPA SYBR Fast qPCR kit (KAPA Biosystems) and either ABI 7300 or StepOnePlus real-time PCR system (Applied Biosystems). Relative abundance of mRNA was calculated by the ΔΔC t method. The mean values of hypoxanthine phosphoribosyltransferse 1 and β-actin are used as normalization controls. The primer pairs used for mouse Ctgf were 5′- CACTCTGCCAGTGGAGTTCA -3′ and 5′- TTACGCCATGTCTCCGTACA -3′; for mouse Birc5 , 5′- TGGCAGCTGTACCTCAAGAA -3′ and 5′- AAAACACTGGGCCAAATCAG -3′; for mouse Inhba , 5′- CATCTTTCCAGTGTCCAGCA -3′ and 5′- CTTCTTCCCATCTCCATCCA -3′; for mouse Mcl1 , 5′- TAACAAACTGGGGCAGGATT -3′ and 5′- AGTCCCGTTTCGTCCTTACA -3′; for mouse Nedd4 , 5′- CATGTGTGGTCTGGGAGATG -3′ and 5′- CCAGAACCAGTGGATGACCT -3′; for mouse Lats2 , 5′- TGAGACAGGACAGCATGGAG -3′ and 5′- ATTTGGTGTCCCGACAAGAG -3′; for mouse WW45 , 5′- GACACGTACCAGGGAATGCT -3′ and 5′- ATACCACTGCTGCCTCTGCT -3′. Reporter assays and cell proliferation assay For reporter assays, HEK293T cells were transfected with indicated plasmids and a β-gal construct plus either TOPflash or FOPflash luciferase reporter. The FOPflash reporter plasmid was used as a negative control. Luciferase activity was measured in a luminometer with a luciferase system (Promega) 24 h post transfection and normalized to β-galactosidase activity. Values are expressed as mean±s.e.m. from three independent experiments. For the cell proliferation assay, NEDD4-KD NIH3T3 cells (1 × 10 4 ) were plated into 35-mm culture dishes. The number of cells was counted everyday for a period of 6 days after plating. Values are expressed as mean±s.e.m. from three independent experiments. Assay for epithelial cell renewal programme Adult flies (5-day-old) were orally administered 5% sucrose solution containing E. carotovora as described previously [60] . To visualize ISC differentiation (EB accumulation), flies carrying Su(H)Gbe-LacZ were used at 16 h post-infection as described previously [60] . Dissected guts were incubated with primary antibodies (anti-PH3 antibody (1:1,000 dilution; Millipore) or anti-LacZ (1:1,000 dilution; Cappel)). Alexa Fluor 568 goat anti-rabbit IgG was used as the secondary antibody. The immunostaining procedure was carried out exactly as described previously [60] . Statistical analysis Values are presented as mean±s.e.m. from at least three to five independent biological replicate experiments with three independent repeated measurements. Data are evaluated by two-tailed one-way analysis of variance with Bonferroni’s post-hoc analysis for multiple comparisons, unless otherwise noted. Statistical calculations were carried out using Prism 5 (GraphPad). P <0.05 was considered statistically significant. How to cite this article : Bae, S. J. et al . NEDD4 controls intestinal stem cell homeostasis by regulating the Hippo signalling pathway. Nat. Commun. 6:6314 doi: 10.1038/ncomms7314 (2015).